Genetically prolonged beige fat in male mice confers long-lasting metabolic health A potential therapeutic target to curb obesity and diabetes is thermogenic beige adipocytes. However, beige adipocytes quickly transition into white adipocytes upon removing stimuli. Here, we define the critical role of cyclin dependent kinase inhibitor 2A (Cdkn2a) as a molecular pedal for the beige-to-white transition. Beige adipocytes lacking Cdkn2a exhibit prolonged lifespan, and male mice confer long-term metabolic protection from diet-induced obesity, along with enhanced energy expenditure and improved glucose tolerance. Mechanistically, Cdkn2a promotes the expression and activity of beclin 1 (BECN1) by directly binding to its mRNA and its negative regulator BCL2 like 1 (BCL2L1), activating autophagy and accelerating the beige-to-white transition. Reactivating autophagy by pharmacological or genetic methods abolishes beige adipocyte maintenance induced by Cdkn2a ablation. Furthermore, hyperactive BECN1 alone accelerates the beige-to-white transition in mice and human. Notably, both Cdkn2a and Becn1 exhibit striking positive correlations with adiposity. Hence, blocking Cdkn2a -mediated BECN1 activity holds therapeutic potential to sustain beige adipocytes in treating obesity and related metabolic diseases. Obesity and its associated metabolic diseases, resulting from chronic energy imbalance, have rapidly prevailed over the past decades worldwide and have become a global public health issue [1] . In mammals, adipocytes are an important regulator of energy homeostasis by storing and releasing energy. White adipocytes store energy as one large lipid droplet, while brown adipocytes with multilocular lipid droplets and abundant mitochondria can dissipate energy to produce heat mediated by uncoupling protein (UCP1) [2] . Notably, beige adipocytes are a subset of “brown-like” cells in white adipose tissue (WAT) that also express UCP1 and contain plentiful mitochondria, thereby possessing thermogenic capability [3] . Although brown adipocytes are limited to infants, beige adipocytes can be recruited throughout WAT by various mechanisms in adult humans, which confers metabolic benefits, including reduced blood glucose and increased energy expenditure [4] , [5] , [6] . Thus, beige adipocytes have emerged as a promising cellular target as a metabolic sink for glucose and free fatty acids to combat obesity and diabetes. In both rodents and humans, the biogenesis of beige adipocytes is highly inducible by a list of physiological and pharmacological stimuli, such as chronic cold exposure or β3 adrenergic receptor agonists [7] . However, beige adipocytes are short-lived; after removing external stimuli, UCP1 + multilocular beige adipocytes convert into dormant unilocular “white” adipocytes, expressing several white adipocyte-enriched genes [8] , [9] , [10] , [11] . Thus, constant stimuli are needed to maintain the activity of beige adipocytes, which has become one of the major clinical hurdles for using beige adipocytes as a sustainable therapy for chronic metabolic diseases. Compared to beige adipocyte triggering, relatively little research has been conducted to investigate the fates of beige adipocytes after discontinuing beiging stimuli. Therefore, it is critical to elucidate the precise mechanism(s) by which beiging is maintained and to examine whether maintaining beiging can improve metabolic fitness. The genomic Cdkn2a locus encodes two crucial cell cycle regulators, p16 Ink4a and p14 ARF , which regulate the p16 Ink4a /RB and p14 ARF /p53 pathways, respectively. The role of Cdkn2a as a tumor suppressor gene is well known [12] , [13] , [14] . Recently, Cdkn2a has been linked to obesity and type 2 diabetes in both rodent and human genome-wide association studies [15] , [16] . Studies have demonstrated that Cdkn2a expression is increased in WAT in obese mouse models and obese humans, inducing senescence and inflammation and aggravating systemic insulin resistance [17] , [18] , [19] . Whole-body Cdkn2a knockout mice gained less weight and fat under a high-fat diet, along with increased beige fat formation in WAT and energy expenditure [19] . Consistent with these studies, our recent study showed that the deletion of Cdkn2a in UCP1-positive cells within inguinal WAT (IGW) stimulated beige adipocyte proliferation [20] . These findings suggest that Cdkn2a plays a crucial role in obesity and diabetes. However, whether Cdkn2a regulates beige fat maintenance is unknown. In this study, we investigated the function of Cdkn2a in beige fat maintenance by employing our defined Cdkn2a mouse models and in vitro beige maintenance assays. We found that loss of Cdkn2a in beige adipocytes results in prolonged beige adipocyte maintenance, enhanced energy expenditure, improved glucose tolerance, and increased resistance to high-fat, high-sucrose (HFHS) diet-induced obesity. Mechanistically, Cdkn2a deficiency promotes beige adipocyte maintenance by inhibiting BECN1-mediated autophagy. Importantly, reactivating autophagy in Cdkn2a -ablated beige adipocytes reversed beige adipocyte maintenance phenotypes. Consistent with a role in energy expenditure, both Cdkn2a and Becn1 exhibit striking positive correlations with adiposity in mice and humans. Collectively, our findings unveil insights into the molecular mechanisms by which Cdkn2a regulates beige adipocyte maintenance via BECN1-mediated autophagy and provide a potential therapeutic strategy to lock into a stable beige identity and treat obesity and related metabolic diseases. Cdkn2a deficiency maintains the morphological and molecular characteristics of beige adipocytes after withdrawal of cold exposure To investigate the function of Cdkn2a in beige fat maintenance in vivo, we crossed tamoxifen (TAM)-inducible Ucp1 -Cre ERT2 mice with a Rosa 26R RFP indelible labeling reporter and Cdkn2a floxed mice ( Cdkn2a Ucp1 KO, Fig. 1a ). Using this fate-mapping model, we first induced beige adipocyte biogenesis in IGW for 7 days by cold exposure (6 °C) to 2-month-old male mice. After cold exposure, we deleted Cdkn2a in all newly induced and preexisting UCP1-expressing beige adipocytes through TAM administration (1.5 mg/kg) for two consecutive days. We housed the mice at room temperature (22 °C) for 60 days (rewarming period) to trace beige adipocyte maintenance (Fig. 1b ). No significant difference was found in body weight or body composition between control and Cdkn2a Ucp1 KO mice after the rewarming period following cold exposure (Fig. 1c and Supplementary Fig. 1a ). As expected, at day 0, all RFP + beige adipocytes within IGW expressed endogenous UCP1 following cold exposure, as assessed by RFP, UCP1, and PLIN immunofluorescence staining (Fig. 1d, e ). Consistent with a previous study that showed that beige adipocytes transition back to their white adipose state [10] , we found that at day 60, nearly 80% of beige adipocytes lost UCP1 expression, as quantified by RFP + , UCP1 − , and PLIN + immunofluorescence staining (Fig. 1d, e ). In contrast, Cdkn2a Ucp1 KO mice contained a higher percentage of UCP1-expressing RFP + beige adipocytes in IGW compared to control mice at 60 days post withdrawal of cold stimulus and TAM administration (Fig. 1d, e ). Consistent with UCP1 immunostaining, hematoxylin and eosin (H&E) staining showed that beige fat biogenesis, determined by multilocular lipids, was similar at day 0 (Fig. 1f ), but Cdkn2a Ucp1 KO mice contained more beige adipocytes at day 60 (Fig. 1g ). Moreover, Cdkn2a deletion reduced adipocyte size in IGW at day 60 (Fig. 1g, h ). At the molecular level, we first confirmed that p16 Ink4 a and p19 Arf , two transcript variants of Cdkn2a , were deleted in IGW beige fat by qPCR analysis (Fig. 1i ). There was no significant difference in the basal expression levels of Ucp1 and other thermogenic genes, such as Ppargc1a , Pparg , and Cidea , in IGW between control and Cdkn2a Ucp1 KO mice at day 0 (Fig. 1i ). In agreement with beige adipocyte maintenance, loss of Cdkn2a increased thermogenic gene expression in IGW at day 60 compared to the control group (Fig. 1j ). Furthermore, we observed a similar pattern of protein abundance of UCP1: no difference at day 0 but significantly higher in IGW from Cdkn2a Ucp1 KO mice after the rewarming period (Fig. 1k ). Similar to the observations in male mice, female Cdkn2a Ucp1 KO mice also exhibited increased beige adipocyte content (Supplementary Data Fig. 1b ) and higher expression levels of thermogenic genes at day 60 compared to control mice (Supplementary Data Fig. 1c ). This suggests that Cdkn2a knockout promotes beige adipocyte maintenance in both male and female mice. To investigate whether increased sympathetic neural signaling was responsible for the prolonged beige fat maintenance in Cdkn2a Ucp1 KO mice, we performed western blot against tyrosine hydroxylase (TH), which is a marker of norepinephrine turnover. However, no significant difference in TH expression was observed in IGW between control and Cdkn2a Ucp1 KO mice at day 60 (Fig. 1l ). Fig. 1: Ablation of Cdkn2a maintains beige adipocyte characteristics after the rewarming period following cold exposure. a Scheme of Cdkn2a Ucp1 KO reporter mice used to conditionally knockout Cdkn2a in UCP1 + cells ( Ucp1 -Cre ERT2 ; Rosa 26R RFP ; Cdkn2a fl/fl ) and label with RFP. b Experimental procedure to track beige adipocytes in vivo. Two-month-old UCP1-RFP (control) and Cdkn2a Ucp1 KO male mice were housed under cold conditions for 7 consecutive days to induce beige fat formation. Mice were then administered tamoxifen (TAM) and fed a chow diet at room temperature for 60 days. c Body weight of male control ( n = 6) or Cdkn2a Ucp1 KO mice ( n = 8). d Immunofluorescence staining of UCP1 and RFP in IGW from control or Cdkn2a Ucp1 KO male mice at day 0 and day 60 post withdrawal of cold stimulus. Scale bar, 50 μM. e Quantification of the percentage of RFP+ cells that express endogenous UCP1. f Representative H&E staining images of IGW from control or Cdkn2a Ucp1 KO male mice at day 0 post withdrawal of cold stimulus. Scale bar, 100 μM. g Tile scan of IGW from control or Cdkn2a Ucp1 KO male mice at day 60 post withdrawal of cold stimulus. Scale bar, 100 μM. h Quantification of adipocyte sizes in IGW from control or Cdkn2a Ucp1 KO male mice at day 60 post withdrawal of cold stimulus ( n = 3). i qPCR analysis of the mRNA expression of p16 Ink4a , p19 Arf and thermogenic genes in IGW from control or Cdkn2a Ucp1 KO male mice at day 0 post withdrawal of cold stimulus ( n = 6). j qPCR analysis of the mRNA expression of p16 Ink4a , p19 Arf and thermogenic genes in IGW from control or Cdkn2a Ucp1 KO male mice at day 60 post withdrawal of cold stimulus ( n = 6). k Western blot analysis of UCP1 in IGW from control or Cdkn2a Ucp1 KO male mice at day 0 and 60 post withdrawal of cold stimulus ( n = 3). l Western blot analysis of TH in IGW from control or Cdkn2a Ucp1 KO male mice at day 60 post withdrawal of cold stimulus ( n = 3). p values were determined by two-tailed Student’s t test. Data are expressed as means ± SEM. Full size image We next evaluated whether deleting Cdkn2a in UCP1 + cells impacted the morphological and molecular characteristics of brown adipocytes and other organs. We observed no differences in interscapular brown adipose tissue (BAT) morphology between control and Cdkn2a Ucp1 KO mice based on H&E analysis (Supplementary Fig. 1d ). In contrast to beige adipocytes, brown adipocytes from both control and Cdkn2a Ucp1 KO mice expressed constitutively high levels of UCP1 even at 60 days after the rewarming period following cold exposure (Supplementary Fig. 1e–g ), which was consistent with a previous study [10] . Moreover, with qPCR analysis, we confirmed that Cdkn2a ( p16 Ink4 a and p19 Arf ) was largely ablated in BAT as expected, while thermogenic gene expression in BAT did not change compared to the control and Cdkn2a Ucp1 KO mice at both day 0 and day 60 (Supplementary Fig. 1h ). Furthermore, morphology and adipocyte size of perigonadal WAT (PGW) showed no significant difference between control and Cdkn2a Ucp1 KO mice (Supplementary Fig. 1i, j ). In addition, no significant difference was observed in liver histology (Supplementary Fig. 1k ) and other tissue weights (Supplementary Fig. 1l ) between control and Cdkn2a Ucp1 KO mice. Overall, these results indicate that Cdkn2a promotes beige adipocyte maintenance but does not affect brown adipocytes or other organs after the rewarming period following cold exposure. Deleting Cdkn2a prevents HFHS-induced obesity and glucose intolerance by enhancing energy expenditure and thermogenesis In both mice and humans, beige adipocytes can reduce body fat and glucose [21] , presenting a key therapeutic promise. Our data thus far suggest that deleting Cdkn2a in beige adipocytes can extend their lifespan but without significant metabolic benefits under a standard chow diet. Chronic exposure to the HFHS diet, which mimics the human diet in many countries, can cause obesity, T2DM, and associated metabolic syndrome [22] . To further understand the functional relevance of Cdkn2a -mediated beige adipocyte maintenance in obesity and its related diabetes, we challenged the control and Cdkn2a Ucp1 KO mice with a HFHS diet for 120 days during the rewarming period following cold exposure (Fig. 2a ). Deleting Cdkn2a prevented HFHS-induced weight gain (Fig. 2b, c ), while food intake showed no significant difference between control and Cdkn2a Ucp1 KO mice (Supplementary Fig. 2a ). Compared to control mice, Cdkn2a Ucp1 KO mice exhibited markedly reduced body fat content and increased lean mass content (Fig. 2d ). Furthermore, Cdkn2a deficiency mainly decreased the weight of WAT depots (IGW, PGW, retroperitoneal WAT (rpWAT)) but not the weight of other tissues, including BAT, muscle, kidney, spleen, pancreas, heart, and liver (Supplementary Fig. 2b ). Cdkn2a knockout decreased adipocyte size in IGW (Fig. 2e, f ) and PGW (Supplementary Fig. 2c, d ). Furthermore, we found that Cdkn2a knockout ameliorated HFHS-induced whitening of BAT (Supplementary Fig. 2e ) and fatty liver (Supplementary Fig. 2e ). Compared to control mice, Cdkn2a Ucp1 KO mice exhibited significantly decreased blood glucose levels (Fig. 2g ) and serum insulin concentrations (Fig. 2h ) under HFHS conditions. Importantly, loss of Cdkn2a improved glucose metabolism and insulin sensitivity compared to control mice, as assessed by the glucose tolerance test (Fig. 2i, j ) and insulin tolerance test (Fig. 2k, l ). Taken together, these results indicate that prolonged maintenance of beige adipocytes by deleting Cdkn2a prevents HFHS-induced body weight and fat mass gain and its associated impaired glucose metabolism. Fig. 2: Prolonged maintenance of beige fat by deleting Cdkn2a prevents HFHS-induced obesity and glucose intolerance by enhancing energy expenditure. a Experimental procedure. Two-month-old UCP1-RFP (control) and Cdkn2a Ucp1 KO male mice were housed under cold conditions for 7 consecutive days to induce beige fat formation. Mice were then administered TAM and fed a HFHS diet at room temperature for 120 days. b Representative images of 6-month-old control or Cdkn2a Ucp1 KO male mice under HFHS. c Body weight of control ( n = 13) or Cdkn2a Ucp1 KO male mice under HFHS ( n = 10). d NMR analysis of fat (left panel) and lean masses (right panel) of body weight of control or Cdkn2a Ucp1 KO male mice under HFHS ( n = 7–15). e Tile scan of IGW from control or Cdkn2a Ucp1 KO male mice under HFHS. Scale bar, 100 μM. f Quantification of adipocyte sizes in IGW from control ( n = 4) or Cdkn2a Ucp1 KO male mice ( n = 3). g The blood glucose level of control ( n = 13) or Cdkn2a Ucp1 KO male mice ( n = 10) ad libitum feeding with HFHS. h The serum insulin level of control ( n = 14) or Cdkn2a Ucp1 KO ( n = 11) male mice under HFHS. i The blood glucose level of control ( n = 14) or Cdkn2a Ucp1 KO ( n = 11) male mice under HFHS after intraperitoneal injection of glucose for glucose (GTT) tolerance tests. j Area under the curve (AUC) analyses of ( i ). k The blood glucose level of control or Cdkn2a Ucp1 KO mice under HFHS after intraperitoneal injection of insulin for insulin (ITT) tolerance tests ( n = 6). l Area under the curve (AUC) analyses of ( k ). m Energy expenditure of control ( n = 5) or Cdkn2a Ucp1 KO ( n = 7) male mice fed a HFHS. n Body temperature of control or Cdkn2a Ucp1 KO male mice during this experiment ( n = 8). o Immunofluorescence staining of UCP1 and RFP in IGW from control or Cdkn2a Ucp1 KO male mice. Scale bar, 50 μM. p Quantification of the percentage of RFP+ cells that express endogenous UCP1. q qPCR analysis of the mRNA expression of thermogenic genes in IGW from control or Cdkn2a Ucp1 KO male mice ( n = 6). r Western blot analysis of UCP1 in IGW from control or Cdkn2a Ucp1 KO male mice ( n = 3). p values were determined by two-tailed Student’s t test. Data are expressed as means ± SEM. Full size image To further investigate the metabolic significance of retaining beige adipocytes in vivo, we next measured gas exchange and whole-body energy expenditure of control and Cdkn2a Ucp1 KO mice under HFHS in metabolic cages. We found that Cdkn2a Ucp1 KO mice showed increases in oxygen consumption (Supplementary Fig. 2f ), carbon dioxide generation (Supplementary Fig. 2g ), and energy expenditure (Fig. 2m ) compared to control mice during both light and dark cycles. No significant difference was found in locomotor activity between control and Cdkn2a Ucp1 KO mice (Supplementary Fig. 2h ). Consistent with the increased metabolic rate, Cdkn2a Ucp1 KO mice also exhibited a higher core body temperature at room temperature (Fig. 2n ). As expected, the H&E staining results showed that Cdkn2a deletion preserved beige fat identity in IGW (Fig. 2e ). Furthermore, Cdkn2a Ucp1 KO mice contained a higher percentage of UCP1-expressing RFP + cells in IGW than control mice (Fig. 2o, p ). Consistently, loss of Cdkn2a maintained higher levels of thermogenic gene expression and UCP1 protein expression and decreased mRNA levels of white adipocyte marker genes, such as Adipoq , Fabp4 , and Lep , in IGW (Fig. 2q, r ), indicating that Cdkn2a knockout prevented beige-to-white adipocyte transition. In contrast, there was no significant difference in the expression of UCP1 and other thermogenic genes in BAT between control and Cdkn2a Ucp1 KO mice (Supplementary Fig. 2i–l ). These data indicate that prolonged maintenance of beige adipocytes by Cdkn2a deletion preserves energy expenditure and promotes thermogenesis under HFHS challenges. Cdkn2a negatively regulates beige adipocyte maintenance in vitro To delineate the underlying cellular and molecular mechanisms, we established a cellular system to study beige adipocyte maintenance in vitro. We isolated stromal vascular fraction (SVF) cells from the IGW of TAM-uninduced control and Cdkn2a Ucp1 KO mice and cultured them to produce beige adipocytes in vitro. After Cdkn2a deletion and RFP labeling by 4-hydroxy-tamoxifen (4-OHT) treatment, we withdrew external stimuli by replacing the differentiation medium with DMEM containing 5% bovine serum albumin (BSA) at the initial stage (day 0). Then we determined how many RFP + cells were still beige adipocytes at the final stage (day 4) (Fig. 3a ). We found that the mRNA levels of p16 Ink4 a and p19 Arf were inversely associated with UCP1 levels among brown, beige, and white adipocytes (Supplementary Fig. 3a ). Furthermore, the mRNA levels of p16 Ink4 a and p19 Arf gradually increased after withdrawing external stimuli (Supplementary Fig. 3b ). Together, these data suggest a negative regulatory role of Cdkn2a in beige adipocyte maintenance. Fig. 3: Cdkn2a deficiency promotes beige adipocyte maintenance in vitro. a Schematic illustration of the cellular system of beige adipocyte maintenance. SVF cells isolated from IGW of control or Cdkn2a Ucp1 KO male mice were differentiated into beige adipocytes and treated with 4-OHT to induce gene deletion and RFP labeling. Then, external stimuli were withdrawn by changing the differentiation medium to DMEM containing 5% BSA for 4 days. b Bright field images of control or Cdkn2a Ucp1 KO beige adipocytes during beige adipocyte maintenance. Scale bar, 100 μM. c Immunofluorescence staining of UCP1 and RFP in control and Cdkn2a Ucp1 KO beige adipocytes during beige adipocyte maintenance. Scale bar, 50 μM. d Quantification of RFP+ cells (upper panel) and the percentage of RFP+ cells that express endogenous UCP1 (lower panel) ( n = 6). e qPCR analysis of the mRNA expression of thermogenic genes in control and Cdkn2a Ucp1 KO beige adipocytes during beige adipocyte maintenance. f Western blot analysis of UCP1 in control and Cdkn2a Ucp1 KO beige adipocytes during beige adipocyte maintenance. g Seahorse analysis of oxygen consumption rates (OCR) in control and Cdkn2a Ucp1 KO beige adipocytes during beige adipocyte maintenance ( n = 12). p values were determined by two-tailed Student’s t test. Data are expressed as means ± SEM of triplicate tests. Full size image At the initial stage, both control and Cdkn2a Ucp1 KO cells exhibited similar amounts of multilocular lipid droplet formation and UCP1 expression (Fig. 3b–d ). At the final stage, the number and size of lipid droplets and UCP1 expression were significantly decreased in control cells (Fig. 3b–d ), recapitulating our in vivo system in which RFP + beige adipocytes lose UCP1 expression. In contrast to control cells, Cdkn2a Ucp1 KO beige adipocytes contained more lipid droplets (Fig. 3b ) and a higher percentage of UCP1-expressing RFP + cells (Fig. 3c, d ) at the final stage. Consistently, no difference was found in the basal expression levels of thermogenic genes between control and Cdkn2a Ucp1 KO beige adipocytes at the initial stage (Supplementary Fig. 3c ). In contrast, at the final stage, Cdkn2a Ucp1 KO cells expressed higher levels of thermogenic genes, such as Ucp1 , Ppargc1a , Pparg , Prdm16 , and Cidea , than control cells (Fig. 3e ). Furthermore, the UCP1 protein level was higher in Cdkn2a Ucp1 KO cells after withdrawing external stimuli than in control cells (Fig. 3f ). Consistent with the higher amount of UCP1 + beige adipocytes in Cdkn2a Ucp1 KO, we found that Cdkn2a deficiency promoted basal mitochondrial respiration and maximal mitochondrial respiratory capacity of beige adipocytes at the final stage but not at the initial stage, as assessed by using a seahorse extracellular flux analyzer (Fig. 3g ). Next, we investigated the role of Cdkn2a in regulating brown adipocyte maintenance in vitro by using the same cellular system (Supplementary Fig. 4a ). In contrast to beige maintenance, the expression levels of p16 Ink4 a and p19 Arf were dramatically decreased during brown adipocyte maintenance (Supplementary Fig. 4b ). Interestingly, the size and number of lipid droplets were decreased in both control and Cdkn2a Ucp1 KO brown adipocytes at the final stage (Supplementary Fig. 4c ). No significant change was found between control and Cdkn2a Ucp1 KO brown adipocytes at either the initial or the final stage, based on morphology and UCP1 immunostaining (Supplementary Fig. 4c–e ). Additionally, thermogenic gene expression was similar between the control and Cdkn2a Ucp1 KO cells during brown fat maintenance (Supplementary Fig. 4f, g ). Collectively, these results indicate that loss of Cdkn2a facilitates the maintenance of beige adipocytes, but not brown adipocytes, in vitro. Cdkn2a regulates beige adipocyte maintenance in a cell cycle-independent manner Since Cdkn2a is a well-known cell cycle inhibitor gene, we examined whether Cdkn2a regulated beige adipocyte maintenance in a cell cycle-dependent manner. Our previous study showed that deleting Cdkn2a in UCP1 + cells in IGW promotes beige adipocyte proliferation [20] . To examine directly if the higher number of UCP1-expressing RFP + cells in Cdkn2a Ucp1 KO was derived from increased proliferative events, we first assessed the proliferation of control and Cdkn2a Ucp1 KO cells during beige fat maintenance by bromodeoxyuridine (BrdU) staining. We observed that Cdkn2a knockout did not affect beige adipocyte proliferation in our in vitro cellular system (Supplementary Fig. 5a ). To further rule out the possibility that beige adipocyte maintenance is regulated in a cell cycle-dependent manner, we examined the role of a downstream gene of Cdkn2a , Ccnd1 , which also plays a key role in the regulation of cell cycle. We found that the mRNA level of Ccnd1 was unchanged during the beige-to-white adipocyte transition (Supplementary Fig. 5b ). To further investigate the effect of Ccnd1 -mediated cell cycle progression on beige-to-white adipocyte transition in vitro, we constructed an adipocyte-specific conditional Ccnd1 overexpression (OE) mouse model (Supplementary Fig. 5c, d ). After doxycycline (Dox) treatment, we confirmed that the Ccnd1 expression was significantly higher in Ccnd1 OE beige adipocytes compared to control cells (Supplementary Fig. 5e ). Overexpression of Ccnd1 did not influence beige adipocyte maintenance, as assessed by immunostaining and western blot analysis of UCP1 (Supplementary Fig. 5f, g ). Together, these findings strongly suggest that beige adipocyte maintenance in Cdkn2a Ucp1 KO mice is not primarily mediated by the activation of cell proliferation. Knockout of Cdkn2a promotes beige fat maintenance by inhibiting autophagy A previous study showed that autophagy-induced mitochondrial clearance (mitophagy) plays a key role in regulating the beige-to-white adipocyte transition [10] . Since Cdkn2a has been strongly associated with autophagy in various cell types [23] , [24] , [25] , we examined the relationship between Cdkn2a and autophagy during beige fat maintenance. Compared to control cells, the number of LC3 puncta, a marker of autophagy, was significantly decreased in Cdkn2a Ucp1 KO beige adipocytes after withdrawing external stimuli (Fig. 4a, b ). We also found that autophagy was activated in control beige adipocytes during the beige-to-white fat transition, as determined by an increased LC3-II/LC3-I ratio and decreased SQSTM1/p62 (a protein specifically degraded in lysosomes) (Fig. 4c ). In contrast, Cdkn2a deficiency inhibited autophagy activation at the final stage (Fig. 4c ), and this autophagy inhibition was further boosted by treatment with the lysosomal inhibitor chloroquine (CQ) (Fig. 4d ). By co-staining with Mitotracker and anti-LC3 antibody, we found that a lower level of mitophagy contributed to the higher mitochondrial content in Cdkn2a Ucp1 KO beige adipocytes compared to control cells (Fig. 4e ). In agreement with this result, Cdkn2a knockout led to an increased mtDNA copy number compared to controls (Fig. 4f ). At the molecular level, Cdkn2a Ucp1 KO beige adipocytes exhibited higher protein abundance of mitochondrial markers VDAC and TOMM20 (Fig. 4g ). In addition, the LC3-II/LC3-I ratio was similar in control and Ccnd1 OE beige adipocytes after withdrawing external stimuli (Supplementary Fig. 5f ), suggesting that Ccnd1 does not affect autophagy during beige adipocyte maintenance. These results indicate that loss of Cdkn2a suppresses autophagy during beige adipocyte maintenance. Fig. 4: Cdkn2a deletion promotes beige fat maintenance by inhibiting autophagy. a Immunofluorescence staining of LC3 and RFP in control and Cdkn2a Ucp1 KO beige adipocytes after withdrawing external stimuli. Scale bar, 10 μM. b Quantification of the number of LC3 puncta per cell ( n = 6). c Western blot analysis of LC3, SQSTM1 in control and Cdkn2a Ucp1 KO beige adipocytes during beige adipocyte maintenance. d Western blotting analysis of LC3 in control and Cdkn2a Ucp1 KO beige adipocytes after withdrawing external stimuli and treated with or without 10 μM chloroquine (CQ). e Immunofluorescence staining of MitoTracker and LC3 in control and Cdkn2a Ucp1 KO beige adipocytes after withdrawing external stimuli. Scale bar, 10 μM. f The relative mtDNA copy number in control and Cdkn2a Ucp1 KO beige adipocytes after withdrawing external stimuli. g Western blot analysis of VDAC and TOMM20 in control and Cdkn2a Ucp1 KO beige adipocytes after withdrawing external stimuli. h Experimental procedure. Two-month-old control and Cdkn2a Ucp1 KO male mice were housed under cold conditions for 7 consecutive days to induce beige fat formation and then administered vehicle or 5 mg/kg rapamycin at room temperature for 90 days. i Representative H&E staining images of IGW from control or Cdkn2a Ucp1 KO male mice treated with or without rapamycin. Scale bar, 100 μM. j Immunofluorescence staining of UCP1 and RFP in control and Cdkn2a Ucp1 KO beige adipocytes treated with or without 10 nM rapamycin after withdrawing external stimuli. Scale bar, 50 μM. k Quantification of the percentage of RFP+ cells that express endogenous UCP1. l qPCR analysis of the mRNA expression of thermogenic genes in control and Cdkn2a Ucp1 KO beige adipocytes treated with or without 10 nM rapamycin after withdrawing external stimuli ( n = 3–4). m Western blot analysis of UCP1 and LC3 in control and Cdkn2a Ucp1 KO beige adipocytes treated with or without 10 nM rapamycin after withdrawing external stimuli. n Seahorse analysis of oxygen consumption rates (OCR) in control and Cdkn2a Ucp1 KO beige adipocytes treated with or without 10 nM rapamycin after withdrawing external stimuli ( n = 9–11). p values were determined by two-tailed Student’s t test. Data are expressed as means ± SEM of triplicate tests. Full size image To test whether Cdkn2a regulated beige adipocyte maintenance in an autophagy-dependent manner, we treated control and Cdkn2a Ucp1 KO mice with rapamycin, an autophagy inducer (Fig. 4h ). We found that rapamycin treatment accelerated the beige-to-white adipocyte transition in control mice (Fig. 4i ), indicating a negative correlation between autophagy activation and beige adipocyte maintenance. Moreover, rapamycin treatment blocked the prolonged beige adipocyte maintenance in IGW from the Cdkn2a Ucp1 KO mice (Fig. 4i ). Consistent with the in vivo data, rapamycin treatment in vitro also largely hindered Cdkn2a Ucp1 KO-mediated beige adipocyte maintenance based on the number of UCP1-expressing RFP + cells (Fig. 4j, k ). Furthermore, the upregulated expression of UCP1 and other thermogenic genes in Cdkn2a Ucp1 KO beige adipocytes was restored to the levels of control cells by rapamycin treatment (Fig. 4l, m ). We confirmed that rapamycin treatment induced autophagy as expected in both control and Cdkn2a Ucp1 KO cells, as assessed by an increased LC3-II/LC3-I ratio (Fig. 4m ). Additionally, rapamycin treatment reversed the enhanced oxygen consumption rate induced by Cdkn2a knockout (Fig. 4n ). Together, these in vivo and in vitro results suggest that Cdkn2a deficiency prevents beige-to-white adipocyte transition by suppressing autophagy. Cdkn2a promotes autophagy by increasing Becn1 expression To investigate how CDKN2A affects autophagy, we tested the effect of Cdkn2a knockout on the mRNA levels of autophagy-related genes in vivo and in vitro. We found that Cdkn2a deficiency reduced the gene expression of Becn1 in both IGW and beige adipocytes, while the expression of other autophagy-related genes, including Atg5 , Atg12 , Pink1 , Bnip3 , Bnip3l , and Fundc1 , was unchanged (Fig. 5a and Supplementary Fig. 6a ). The protein expression of BECN1 was increased in the control group after withdrawing external stimuli (Fig. 5b and Supplementary Fig. 6b ). Compared to the control group, the Cdkn2a knockout group exhibited lower protein levels of BECN1 in vivo and in vitro (Fig. 5b and Supplementary Fig. 6b ). Furthermore, we found that the mRNA level of Becn1 was significantly higher in IGW than in BAT (Supplementary Fig. 6c ). Consistently, thermogenic brown and beige adipocytes expressed lower Becn1 (Supplementary Fig. 6d ), indicating a negative correlation between Becn1 and thermogenesis. Similar to the expression pattern of p16 Ink4 a and p19 Arf , the gene expression of Becn1 was increased after withdrawing external stimuli (Fig. 5c ). Interestingly, the deletion of Cdkn2a in brown adipocytes also inhibited Becn1 expression in vivo and in vitro (Supplementary Fig. 6e, f ). Fig. 5: Cdkn2a regulates autophagy by positively mediating Becn1 expression in vivo and in vitro. a qPCR analysis of the mRNA expression of autophagy-related genes in IGW from control or Cdkn2a Ucp1 KO male mice fed a HFHS ( n = 6). b Western blot analysis of BECN1 in IGW from control or Cdkn2a Ucp1 KO male mice. c Expression profile of Becn1 during beige adipocyte maintenance. d Experimental procedure. Two-month-old control, Cdkn2a Ucp1 KO and Cdkn2a Ucp1 KO + Becn1 F121A male mice were housed under cold conditions for 7 consecutive days to induce beige fat formation. Mice were then administered tamoxifen (TAM) and fed a chow diet at room temperature for 20 days. e Representative H&E staining images of IGW from control, Cdkn2a Ucp1 KO or Cdkn2a Ucp1 KO + Becn1 F121A male mice after cold stimulus withdrawal. Scale bar, 100 μM. f Immunofluorescence staining of UCP1 in IGW from control, Cdkn2a Ucp1 KO or Cdkn2a Ucp1 KO + Becn1 F121A male mice after cold stimulus withdrawal. Scale bar, 50 μM. g Quantification of the percentage of RFP+ cells that express endogenous UCP1. h qPCR analysis of the mRNA expression of thermogenic genes in IGW from control, Cdkn2a Ucp1 KO or Cdkn2a Ucp1 KO + Becn1 F121A male mice after cold stimulus withdrawal ( n = 6). i Western blot analysis of UCP1 and LC3 in IGW from control, Cdkn2a Ucp1 KO or Cdkn2a Ucp1 KO + Becn1 F121A male mice after cold stimulus withdrawal. j Immunofluorescence staining of UCP1 and RFP in control and Cdkn2a Ucp1 KO beige adipocytes with or without hyperactive BECN1 after withdrawing external stimuli. Scale bar, 50 μM. k Quantification of the percentage of RFP+ cells that express endogenous UCP1. l qPCR analysis of the mRNA expression of thermogenic genes in control and Cdkn2a Ucp1 KO beige adipocytes with or without hyperactive BECN1 after withdrawal of external stimuli ( n = 4–6). m Western blot analysis of UCP1 and LC3 in control and Cdkn2a Ucp1 KO beige adipocytes with or without hyperactive BECN1 after withdrawing external stimuli. p values were determined by two-tailed Student’s t test. Data are expressed as means ± SEM of triplicate tests. Full size image To test whether Cdkn2a within beige adipocytes regulated autophagy via Becn1 , we performed in vitro beige maintenance assays using a previously established hyperactive BECN1 mouse model induced by a single knock-in mutation (F121A) that decreases its interaction with the negative regulator BCL2 [26] (Supplementary Fig. 6g ). We examined whether Cdkn2a Ucp1 KO beige adipocytes could still be maintained in a hyperactive BECN1 setting (Fig. 5d ). After a short 20-day rewarming period following cold exposure, we found that hyperactive BECN1 blunted Cdkn2a Ucp1 knockout--mediated beige adipocyte maintenance based on H&E analysis (Fig. 5e ). We further performed RFP and UCP1 immunostaining on IGW sections and confirmed that upon hyperactive BECN1 ( Cdkn2a Ucp1 KO + Becn1 F121A ), Cdkn2a Ucp1 KO beige adipocytes started to lose UCP1 expression at day 20 of the rewarming period, with a similar percentage of UCP1-expressing RFP + cells (Fig. 5f, g ) and comparable levels of thermogenic gene expression within IGW (Fig. 5h, i ) as the control group. In agreement with these mouse models, we confirmed that the autophagy level was restored to the control level in Cdkn2a Ucp1 KO+ Becn1 F121A mice compared to control and Cdkn2a Ucp1 KO mice (Fig. 5i ), as determined by western blot analysis of the LC3-II/LC3-I ratio. Consistent with our in vivo data, hyperactive BECN1 also impaired Cdkn2a knockout-mediated beige adipocyte maintenance in vitro, as assessed by quantification of UCP1-expressing RFP + cells (Fig. 5j, k ). Additionally, the mRNA expression of UCP1 and other thermogenic genes in the Cdkn2a Ucp1 KO beige adipocytes was restored to the levels in the control mice after hyperactive BECN1 (Fig. 5l, m ). Together, these findings suggest that Cdkn2a regulates beige adipocyte maintenance through BECN1-mediated autophagy. Hyperactive BECN1 accelerates the loss of beige adipocyte characteristics upon removal of external stimuli in vitro To investigate the role of BECN1 in beige fat maintenance, we isolated SVF cells from Becn1 F121A mice and performed in vitro studies (Fig. 6a ). We first confirmed that hyperactive BECN1 increased the number of LC3 puncta and the LC3-II/LC3-I ratio, hallmarks of enhanced autophagy, in beige adipocytes compared to control cells (Fig. 6b–d ). We found that hyperactive BECN1 did not affect beige adipogenesis (Fig. 6e, f ) or UCP1 expression at the initial stage (day 0) (Fig. 6g, h ). At the final stage (day 2), hyperactive BECN1 impaired beige adipocyte maintenance and decreased thermogenic gene expression (Fig. 6g–j ). We also investigated the function of BECN1 in brown adipocyte maintenance (Supplementary Fig. 7a ). Hyperactive BECN1 also enhanced autophagy in brown adipocytes (Supplementary Fig. 7b, c ) but did not affect brown fat biogenesis (Supplementary Fig. 7d, e ). Similar to Cdkn2a knockout in beige adipocytes, no significant difference was observed in maintenance or thermogenic gene expression between control and Becn1 F121A brown adipocytes at the final stage (Supplementary Fig. 7f–h ), suggesting that BECN1-promoted autophagy was not a regulator of brown adipocyte maintenance. Together, these findings suggest that hyperactive BECN1 impairs the maintenance of beige adipocytes but not brown adipocytes. Fig. 6: BECN1 does not influence beige biogenesis but accelerates the loss of beige adipocyte characteristics after withdrawal of external stimuli in vitro. a Schematic illustration of the cellular system of beige adipocyte maintenance. SVF cells isolated from IGW of control or Becn1 F121A male mice were differentiated into beige adipocytes. Then, external stimuli were withdrawn by changing the differentiation medium to DMEM containing 5% BSA for 2 days. b Immunofluorescence staining of LC3 in control and Becn1 F121A beige adipocytes. Scale bar, 10 μM. c Quantification of the number of LC3 puncta per cell ( n = 6). d Western blot analysis of LC3 in control and Becn1 F121A beige adipocytes. e Oil red O staining of control and Becn1 F121A beige adipocytes before withdrawing external stimuli. Scale bar, 100 μM. f Relative lipid accumulation was quantified with a microplate spectrophotometer. g Immunofluorescence staining of UCP1 and PLIN1 in control and Becn1 F121A beige adipocytes during beige adipocyte maintenance. Scale bar, 50 μM. h Quantification of the percentage of UCP1-expressing cells ( n = 6). i qPCR analysis of the mRNA expression of thermogenic genes in control and Becn1 F121A beige adipocytes during beige adipocyte maintenance. j Western blot analysis of UCP1 in control and Becn1 F121A beige adipocytes during beige adipocyte maintenance. k Western blot analysis of UCP1 and LC3 in human beige adipocytes treated with or without 5 μM Tat-BECN1 after withdrawal of external stimuli. l qPCR analysis of the mRNA expression of thermogenic genes in human beige adipocytes treated with or without 5 μM Tat-BECN1 after withdrawal of external stimuli. p values were determined by two-tailed Student’s t test. Data are expressed as means ± SEM of triplicate tests. Full size image To further investigate whether BECN1-mediated autophagy regulates human beige adipocyte maintenance, we isolated SVF cells from human subcutaneous WAT and performed in vitro beige maintenance assays. We induced human beige adipogenesis and treated cells with Tat-Becn1, a peptide known to stimulate autophagy through the mobilization of endogenous BECN1 [27] , after the withdrawal of stimuli. We validated that Tat-Becn1 enhanced autophagy in human beige adipocytes, as assessed by an increased LC3-II/LC3-I ratio (Fig. 6k ). As expected, Tat-BENC1 accelerated the decrease of expression of UCP1 and other thermogenic genes in human beige adipocytes after removing stimuli (Fig. 6k, l ). These results indicate that BECN1-mediated autophagy plays a conserved role in regulating beige adipocyte maintenance between humans and mice. p16 INK4a facilitates Becn1 expression by preventing its mRNA decay To explore the underlying mechanisms by which Cdkn2a regulates BECN1-mediated autophagy in beige adipocytes, we first examined whether there were any changes in the cellular distributions of p16 INK4a and p19 ARF during the beige-to-white transition. Intriguingly, the cytoplasmic accumulation of p16 INK4a in beige adipocytes was significantly increased 6 h post withdrawing external stimuli, while the cellular distribution of p19 ARF was unaltered (Fig. 7a ), suggesting that p16 INK4a and p19 ARF might play distinct roles in mediating Becn1 . Since a previous mRNA-bound proteome study identified p16 INK4a and p19 ARF as potential RNA-binding proteins [28] , we decided to investigate whether p16 INK4a and/or p19 ARF regulate Becn1 expression by binding to its mRNA. We performed RNA immunoprecipitation (RIP)-qPCR with antibodies against endogenous p16 INK4a or p19 ARF (Fig. 7b ). We found that p16 INK4a interacted with the mRNA of Becn1 , but not Atg5 , Atg7 , Pink1 , or Ucp1 , in beige adipocytes upon withdrawal of external stimuli (Fig. 7c ). In addition, no interaction was observed between p19 ARF and Becn1 mRNA (Fig. 7d ). Together, these results indicate that p16 INK4a regulates Becn1 by specifically targeting its transcript. Fig. 7: Cdkn2a positively regulates Becn1 expression by suppressing its mRNA decay and promotes BECN1-mediated autophagy by interacting with BCL2L1. a Immunofluorescence staining of p16 INK4a and p19 ARF distribution during beige adipocyte maintenance. b Western blot to confirm the immunoprecipitation of p16 INK4a and p19 ARF proteins. c RNA immunoprecipitation-qPCR (RIP-qPCR) analysis of the interaction of Becn1 , Atg5 , Atg12 , Pink1 and Ucp1 transcripts with p16 INK4a in beige adipocytes ( n = 3). d RNA immunoprecipitation-qPCR (RIP-qPCR) analysis of the interaction of the Becn1 transcript with p19 ARF in beige adipocytes ( n = 3). e mRNA lifetimes of Becn1 and Ucp1 in control and Cdkn2a Ucp1 KO beige adipocytes ( n = 3). f Co-immunoprecipitation (Co-IP) analysis of the interaction between p19 ARF and BECN1 or BCL2L1. g Co-IP analysis of the interaction between p16 INK4a and BECN1 or BCL2L1. h Co-IP analysis of the interaction between BCL2L1 and BECN1 in control and Cdkn2a Ucp1 KO beige adipocytes after withdrawing external stimuli ( n = 3). Quantification of the BECN1/BCL2L1 ratio in the IP samples is shown in the right panel. i Working model. In wild type cells, p16 INK4a specifically targets Becn1 mRNA and increases its expression by promoting mRNA stability, while p19 ARF interacts with BCL2L1 and releases BECN1, thereby enhancing autophagy and beige-to-white transition. Loss of Cdkn2a decreases the protein levels of p16 INK4a and p19 ARF , resulting in reduced expression and activity of BECN1, thereby inhibiting autophagy and promoting beige fat maintenance. p values were determined by two-tailed Student’s t test. Data are expressed as means ± SEM. Full size image Since p16 INK4a positively modulated Becn1 gene expression and p16 INK4a was involved in the regulation of mRNA stability [29] , we investigated the Becn1 mRNA stability in control and Cdkn2a Ucp1 KO beige adipocytes by using an RNA decay assay. As expected, Cdkn2a deficiency markedly decreased the mRNA stability of Becn1 , but not Ucp1 , in beige adipocytes (Fig. 7e ). Collectively, these results demonstrate that p16 INK4a serves as an RNA-binding protein during the beige-to-white transition and regulates Becn1 expression by mediating its mRNA stability. p19 ARF promotes BECN1-mediated autophagy by interacting with BCL2L1 A previous study reported that p19 ARF reduced the formation of the protein complex between BECN1 and its negative regulator, BCL2L1, and then induced autophagy in cancer cells [23] . Here, we asked whether p19 ARF might interfere with the ability of BCL2L1 to complex with BECN1 protein, leading to enhanced autophagy during the beige-to-white transition. To test this hypothesis, we first detected the interaction among p19 ARF , BECN1 and BCL2L1 in beige adipocytes. Using a co-IP assay, we found that p19 ARF could interact with BECN1 and BCL2L1 (Fig. 7f ). In contrast, p16 INK4a was unable to interact with BECN1 or BCL2L1 (Fig. 7g ). In the reciprocal IP, p19 ARF was also pulled down by an antibody against BCL2L1 (Fig. 7h ). Importantly, the complex formation between BECN1 and BCL2L1 was markedly increased in Cdkn2a Ucp1 KO beige adipocytes compared to control cells (Fig. 7h ). Taken together, these results indicate that p19 ARF enhances BECN1-mediated autophagy by interacting with BCL2L1. Cdkn2a and Becn1 expression are positively associated with obesity in mice and humans We further investigated the correlation between Cdkn2a and Becn1 mRNA levels and obesity. Upon HFHS feeding, the mRNA levels of p16 Ink4 a , p19 Arf , and Becn1 in IGW were significantly higher than in mice fed a standard chow diet (Fig. 8a ). Most remarkably, the p16 INK4 a , p14 ARF , and BECN1 mRNA levels in subcutaneous adipose tissues of obese human individuals were significantly higher than that of non-obese individuals (Fig. 8b ), linking p16 INK4 a , p14 ARF , and BECN1 expression to obesity in human. Furthermore, we found that higher mRNA levels of p16 INK4 a and p14 ARF were associated with higher body weight, BMI, and fat mass in humans (Fig. 8c, d ). BECN1 expression was positively correlated with body weight, BMI, fat mass, and blood glucose levels (Fig. 8e ). Thus, these data indicate that CDKN2A and BECN1 mRNA levels could be indicators of human obesity and T2DM. Fig. 8: Cdkn2a and Becn1 expression levels positively correlate with obesity in mice and humans. a qPCR analysis of the mRNA expression of p16 Ink4a , p19 Arf and Becn1 in IGW from male mice fed on chow diet or HFHS ( n = 6–7). b qPCR analysis of the mRNA expression of p16 Ink4a , p14 Arf and Becn1 in subcutaneous WAT from obese and non-obese people ( n = 5–12). c Two-tailed Pearson’s correlation analysis of p16 INK4a expression in human subcutaneous WAT and body weight, BMI or fat mass of 17 individuals. d Two-tailed Pearson’s correlation analysis of p14 ARF expression in human subcutaneous WAT and body weight, BMI or fat mass of 17 individuals. e Two-tailed Pearson’s correlation analysis of BECN1 expression in human subcutaneous WAT and body weight, BMI, fat mass and blood glucose levels of 15–17 individuals. p values were determined by two-tailed Student’s t test. Data are expressed as means ± SEM. Full size image Since the rediscovery of brown and beige adipocytes in adults, tremendous efforts have been made to find signals to induce beige adipocyte formation within WAT. In this study, we used unique mouse models to demonstrate that beige adipocytes can be formed and maintained by pharmacological and genetic methods. The main finding of this study is that Cdkn2a is a crucial negative regulator of beige adipocyte maintenance through direct interaction with Becn1 . We report that genetically deleting Cdkn2a in beige adipocytes promotes their lifespan and is associated with an improved metabolic profile upon HFHS diet challenge. Our data reveal a previously unknown function of Cdkn2a in beige fat biology and suggest that inhibitors of the Cdkn2a pathway would be beneficial in reversing the deleterious effects of metabolic syndromes. Therefore, it serves as a potential therapeutic target in treating obesity and its related metabolic diseases. Activation of beige fat biogenesis is accompanied by improved metabolic benefits. There is, however, little evidence that maintaining beige adipocyte phenotype can be beneficial. In this study, we investigated whether sustained beige adipocytes can improve metabolic fitness under diet-induced obesity, thereby achieving anti-obesity and anti-diabetes effects. We found that Cdkn2a deletion promotes beige adipocyte maintenance under both a standard chow and a HFHS diet. Importantly, the retained beige adipocytes, induced by UCP1 + -cell-specific Cdkn2a deletion, are adequate to prevent body weight gain, fat expansion, and ectopic lipid storage in the liver under HFHS feeding. Along with the presence of preserved beige adipocytes, the mice also have improved glucose tolerance. These results are intriguing, given the recent clinical observation that a strong association exists between greater brown fat activity and lower cardiovascular risk, such as high blood pressure and coronary artery disease [30] . Several recent studies have shown that beige and brown fat can influence systemic metabolism through releasing endocrine signals, including peptides, lipids, miRNAs, and secreted proteins, independent of non-shivering thermogenesis [31] , [32] . Our data suggest that signals released from Cdkn2a Ucp1 KO beige adipocytes may communicate with other organs to maintain whole-body energy metabolism. One critical obstacle in beige adipocyte research is that there are no specific Cre lines to precisely target brown vs. beige adipocytes in mouse models. Deletion of Cdkn2a by UCP1-Cre ERT2 inevitably creates a model with gene knockout in brown fat, which may confound the phenotype. However, in our Cdkn2a Ucp1 KO model, we did not observe BAT phenotypes based on morphology and thermogenic gene expression profile, indicating that the resulting metabolic benefits may largely come from beige adipocyte maintenance. Interestingly, although our data suggest that BAT maintenance is independent of Cdkn2a and Becn1 , the regulation of Becn1 expression by Cdkn2a is essentially conserved in brown and beige adipocytes both in vivo and in vitro. It is thus conceivable that, in addition to Cdkn2a and Becn1 , multiple complex mechanisms may exist to retain BAT identity and their physiological roles. Combined with the prior knowledge that beige adipocytes are developmentally, molecularly, and functionally different from brown adipocytes [33] , our finding substantiates this important concept that brown and beige adipocyte identities are different and are also distinctly regulated. Mechanistically, we found that Cdkn2a deficiency mediates beige adipocyte maintenance by regulating autophagy and is independent of Ccnd1 activity and likely independent of cell cycle control. During the beige-to-white transition, autophagy genes have been shown to contribute to beige adipocyte “whitening” [10] , [11] , [34] , [35] , [36] . Interestingly, we found that rapamycin further decreased Ucp1 and Cidea expression compared to the control mice. As rapamycin is an inhibitor of mTORC1, which is essential for promoting beige adipogenesis [37] , [38] , it is possible that rapamycin repressed beige adipocyte activity by inhibiting the mTORC1 pathway. Consistently, early studies using adipose-specific deletion of autophagy-related genes show that mice accumulate more mitochondria in WAT, producing a browning of WAT phenotype with reduced body weight and WAT mass [39] , [40] . Among the autophagy pathway, BECN1 is a scaffolding protein that is key for the initiation of autophagosome biogenesis [41] , and therefore, we can target and activate autophagy at early steps; the role of BECN1 in adipose tissue has been recently appreciated: adipocyte-specific BECN1 knockout mice develop severe lipodystrophy and metabolic dysfunctions [42] , [43] . However, it is not clear what role BECN1 plays in UCP1 + cells and whether BECN1 mediates beige activity downstream of the Cdkn2a pathway. In this study, we identified the Cdkn2a pathway as an upstream mechanism that cooperates with autophagy regulation to govern beige-to-white adipocyte transition. More specifically, p16 INK4a facilitates Becn1 expression by its function in preventing its mRNA decay, and p19 ARF promotes BECN1-mediated autophagy by interacting with its negative regulator BCL2L1. Thus, our findings provide mechanistic insights into key players in beige fat maintenance regulation. Therapeutically, the expressions of both Cdkn2a and Becn1 are upregulated in obesity and positively associated with adiposity in mice and humans. Our findings reveal that Cdkn2a and Becn1 function as potent positive regulators of beige-to-white adipocyte transition, providing a potential therapeutic target for pharmacological intervention to combat the obesity epidemic and its related metabolic diseases. Since direct manipulation of either Cdkn2a or Becn1 could cause several downstream effects and/or potential tumor formation, we believe that defining specific upstream and downstream factors of the Cdkn2a - Becn1 pathway will pave the way to develop more focused treatments for obesity and metabolic diseases. Previously, we and others have demonstrated that the ability to form beige adipocytes declines when mice grow older [44] , [45] , [46] , [47] , [48] , [49] , [50] , [51] . Therefore, it will be interesting to test whether manipulating Cdkn2a or Becn1 still maintains their beiging capacity and whether beige adipocytes can be maintained in the older stage. The possibility that the beiging potential can be retained in obese and aged humans and animals suggests a potential therapeutic approach to use beige adipocytes against obesity in older adults. In summary, we have identified Cdkn2a as an important player in beige adipocyte maintenance via Becn1-mediated autophagy. Our work creates a concept that beige adipocytes can stay long-lived after discontinuing the stimuli and could be developed as an alternative therapeutic target for treating obesity by improved energy expenditure and metabolic fitness. Mouse models Mice were housed at 22 ± 2 °C with a humidity of 35 ± 5% and a 14:10 light:dark cycle with a standard rodent chow diet and water unless otherwise indicated. Rosa26R RFP (Stock No. 007914) mice were obtained from the Jackson Laboratory. Ucp1 -Cre ERT2 and Cdkn2a fl/fl mice were generously provided by Dr. Eric N. Olson (University of Texas Southwestern Medical Center). Becn1 F121A mice were generously provided by Dr. Congcong He (Northwestern University). All mice were maintained on mixed C57BL6/J-129SV background. All animal experiments were performed according to procedures reviewed and approved by the Institutional Animal Care and Use Committee of the University of Illinois at Chicago. Mice were euthanized by carbon dioxide asphyxiation (CO 2 ) inhalation and cervical dislocation was performed as a secondary euthanasia procedure. Generation of TRE-Ccnd1 mice Mice were generated as previously described [52] . Briefly, we introduced p2Lox- Ccnd1 into ZX1 ES cells and selected for G418-resistant recombinant colonies, in which Ccnd1 was recombined downstream of a tetracycline-responsive promoter (TRE). ZX1 ES cell clones were then validated in culture, and three clones were used to generate three chimeric mouse lines. All three-mouse strains (TRE- Ccnd1 ) behaved similarly and had similar induction of Ccnd1 expression in response to doxycycline. Cell culture The isolated cells were cultured in DMEM/F12 media (Sigma-Aldrich) supplemented with 10% FBS (Sigma-Aldrich) and 1% Penicillin/Streptomycin (Gibco) at 37 °C in a 5% CO 2 humidified incubator. For beige and brown adipocyte differentiation, post-confluent cells were induced by DMEM/F12 containing 10% FBS, 0.5 mM isobutylmethylxanthine (Sigma-Aldrich), 1 µg/ml insulin (Sigma-Aldrich), 1 µM dexamethasone (Sigma-Aldrich), 60 µM indomethacin (Sigma-Aldrich), 1 nM triiodo-L-thyronine (Sigma-Aldrich), and 1 µM rosiglitazone (Sigma-Aldrich) for 2 days and with DMEM/F12 containing 10% FBS and 1 µg/ml insulin, 1 nM triiodo-L-thyronine, and 1 µM rosiglitazone every 2 days. Fresh medium was replaced every 2 days until ready for harvest. To withdraw external stimuli, the differentiation medium was changed to DMEM containing 5% BSA for 4 days. Tamoxifen treatment To induce Cre recombination, mice were intraperitoneally injected with 1.5 mg/kg body weight of tamoxifen (TAM; Cayman Chemical) dissolved in sunflower oil (Sigma-Aldrich) for 2 consecutive days. For Cre induction in vitro, cells were treated with 2 µM 4-hydroxy-Tamoxifen (4-OHT, Sigma-Aldrich). Cold exposure experiment For cold exposure experiments, mice were placed in a 6 °C environmental chamber (Environmental & Temperature Solutions) for 7 days. Body temperature was measured using a rectal probe (Physitemp). The probe was lubricated with glycerol and inserted 1.27 centimeters (0.5 inch), and the temperature was recorded when stabilized at the indicated time points. Metabolic cage studies Mice were housed individually and acclimatized to the metabolic chambers (Promethion System, Sable System International) at the UIC Biologic Resources Laboratory for 2 days before data collection was initiated. For the subsequent 3 days, food intake, VO 2 , VCO 2 , energy expenditure and physical activity were monitored over a 12 h light/dark cycle with food provided ad libitum. For energy expenditure analysis, embedded ANCOVA tools in a web application CalR [53] were used to perform regression-based indirect calorimetric analysis. For body composition analysis, the total fat and lean mass were assessed with Bruker Minispec 10 whole body composition analyzer (Bruker). Glucose and insulin tolerance tests For the glucose tolerance test, mice fasted for 16 h were intraperitoneally injected with glucose (1.5 g/kg). For insulin tolerance test, mice fasted for 4 h were intraperitoneally injected with human insulin (1.0 U/kg). Glucose levels were measured in tail blood at 0, 15, 30, 45, 60, 90 and 120 min after glucose injection by using a glucose meter (Contour Next). Isolation of stromal vascular fraction (SVF) Isolation of SVF cells from IGW and BAT was performed as previously described [20] . Briefly, IGW or BAT was excised from 6-week-old male mice, minced by scissors and then digested in isolation buffer (100 mM HEPES, 0.12 M NaCl, 50 mM KCl, 5 mM D-glucose, 1.5% BSA, 1 mM CaCl 2 , pH 7.3) containing 1 mg/ml type I collagenase (Worthington) at 37 °C for 30 min. Digested tissue was filtered through 70 µm mesh to remove large pieces, and the flow-through was then centrifuged at 800 × g for 5 min. Pellets containing primary preadipocytes were resuspended in red blood cell lysis buffer (155 mM NH 4 Cl, 10 mM KHCO 3 , 0.1 mM EDTA) for 5 min, followed by centrifugation at 800 × g for 5 min. The pellets were resuspended and seeded. Human SVF cells were isolated from fresh subcutaneous adipose tissues. Western blot analysis Proteins from cells and tissue were extracted with RIPA buffer (Boston BioProducts) supplemented with protease inhibitor cocktail (MedChem Express) and centrifuged at 12,000 × g for 15 min at 4 °C. The total protein amounts were detected by a BCA assay kit (Thermo Fisher Scientific). Protein samples were separated in an SDS-PAGE gel and transferred to PVDF membranes (Millipore). The membranes were blocked with 5% non-fat milk at room temperature and then incubated with relevant primary antibodies at 4 °C overnight, followed by HRP-conjugated secondary antibody at room temperature for 2 h. The signals were detected by the addition of Western ECL Substrate (Thermo Fisher Scientific). The protein bands were detected using ChemiDoc MP Image system (Biorad). 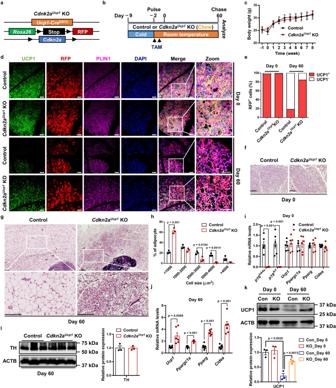Fig. 1: Ablation ofCdkn2amaintains beige adipocyte characteristics after the rewarming period following cold exposure. aScheme ofCdkn2aUcp1KO reporter mice used to conditionally knockoutCdkn2ain UCP1+cells (Ucp1-CreERT2;Rosa26RRFP;Cdkn2afl/fl) and label with RFP.bExperimental procedure to track beige adipocytes in vivo. Two-month-old UCP1-RFP (control) andCdkn2aUcp1KO male mice were housed under cold conditions for 7 consecutive days to induce beige fat formation. Mice were then administered tamoxifen (TAM) and fed a chow diet at room temperature for 60 days.cBody weight of male control (n= 6) orCdkn2aUcp1KO mice (n= 8).dImmunofluorescence staining of UCP1 and RFP in IGW from control orCdkn2aUcp1KO male mice at day 0 and day 60 post withdrawal of cold stimulus. Scale bar, 50 μM.eQuantification of the percentage of RFP+ cells that express endogenous UCP1.fRepresentative H&E staining images of IGW from control orCdkn2aUcp1KO male mice at day 0 post withdrawal of cold stimulus. Scale bar, 100 μM.gTile scan of IGW from control orCdkn2aUcp1KO male mice at day 60 post withdrawal of cold stimulus. Scale bar, 100 μM.hQuantification of adipocyte sizes in IGW from control orCdkn2aUcp1KO male mice at day 60 post withdrawal of cold stimulus (n= 3).iqPCR analysis of the mRNA expression ofp16Ink4a,p19Arfand thermogenic genes in IGW from control orCdkn2aUcp1KO male mice at day 0 post withdrawal of cold stimulus (n= 6).jqPCR analysis of the mRNA expression ofp16Ink4a,p19Arfand thermogenic genes in IGW from control orCdkn2aUcp1KO male mice at day 60 post withdrawal of cold stimulus (n= 6).kWestern blot analysis of UCP1 in IGW from control orCdkn2aUcp1KO male mice at day 0 and 60 post withdrawal of cold stimulus (n= 3).lWestern blot analysis of TH in IGW from control orCdkn2aUcp1KO male mice at day 60 post withdrawal of cold stimulus (n= 3).pvalues were determined by two-tailed Student’sttest. Data are expressed as means ± SEM. The primary antibodies used in this study are listed in Supplementary Table 1 . Histological staining Hematoxylin and eosin (H&E) staining was performed on paraffin sections using standard methods. Briefly, tissues were fixed in 10% formalin overnight, dehydrated, embedded in paraffin, and sectioned with a microtome at 4–8 μm thicknesses. Adipocyte sizes were quantified by using ImageJ. For immunohistochemistry (IHC), sections were deparaffinized, boiled in antigen-retrieval solution, treated with primary antibodies in blocking buffer (5% donkey serum) at 4 °C overnight, treated with secondary antibody for 2 h at room temperature in blocking buffer, and stained with Vectastain ABC KIT (Vector Laboratories) and DAB KIT (Vector Laboratories). Immunostaining images were taken using a Leica DMi8 microscope (Leica). For immunofluorescence staining, paraffin sections were incubated with permeabilization buffer (0.3% Triton X-100 in PBS) for 30 min at room temperature, with primary antibody at 4 °C overnight, and with secondary antibody for 2 h at room temperature, all in blocking buffer (5% donkey serum in 1X PBS). Images were taken using a confocal laser microscope (Carl Zeiss Ltd). Oil red O staining Cells were washed and fixed in 4% paraformaldehyde at room temperature for 1 h. After washing with 60% isopropanol three times, the cells were stained with 60% filtered Oil Red O working solution (vol/vol in distilled water) of Oil red O stock solution (Sigma-Aldrich) at room temperature for 15 min. Cells were washed with ddH 2 O before imaging. To quantify lipid accumulation, Oil Red O-stained lipids were eluted in 100% isopropanol, and then the optical density (OD) was measured at 500 nm. RNA isolation and quantitative real-time PCR (qPCR) analysis Total RNA from tissue or cells was isolated using Tripure Isolation Reagent (Sigma-Aldrich) and Bullet Blender Homogenizer (Next Advance) according to the manufacturer’s protocol. cDNA was converted from 2 μg of total RNA by using a High Capacity cDNA Reverse Transcription Kit (Thermo Fisher Scientific). qPCR was performed using 2X Universal SYBR Green Fast qPCR Mix (Abclonal) following the manufacturer’s instructions and analyzed with a ViiA7 system (Applied Biosystems). Data were analyzed using the comparative Ct method and the relative expression of mRNAs was determined after normalization to Rplp0 . 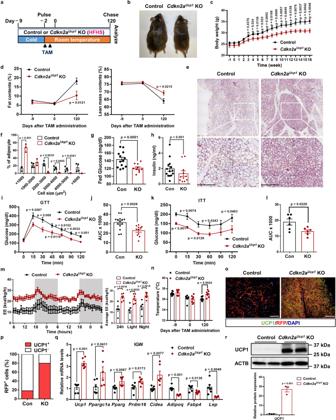Fig. 2: Prolonged maintenance of beige fat by deletingCdkn2aprevents HFHS-induced obesity and glucose intolerance by enhancing energy expenditure. aExperimental procedure. Two-month-old UCP1-RFP (control) andCdkn2aUcp1KO male mice were housed under cold conditions for 7 consecutive days to induce beige fat formation. Mice were then administered TAM and fed a HFHS diet at room temperature for 120 days.bRepresentative images of 6-month-old control orCdkn2aUcp1KO male mice under HFHS.cBody weight of control (n= 13) orCdkn2aUcp1KO male mice under HFHS (n= 10).dNMR analysis of fat (left panel) and lean masses (right panel) of body weight of control orCdkn2aUcp1KO male mice under HFHS (n= 7–15).eTile scan of IGW from control orCdkn2aUcp1KO male mice under HFHS. Scale bar, 100 μM.fQuantification of adipocyte sizes in IGW from control (n= 4) orCdkn2aUcp1KO male mice (n= 3).gThe blood glucose level of control (n= 13) orCdkn2aUcp1KO male mice (n= 10) ad libitum feeding with HFHS.hThe serum insulin level of control (n= 14) orCdkn2aUcp1KO (n= 11) male mice under HFHS.iThe blood glucose level of control (n= 14) orCdkn2aUcp1KO (n= 11) male mice under HFHS after intraperitoneal injection of glucose for glucose (GTT) tolerance tests.jArea under the curve (AUC) analyses of (i).kThe blood glucose level of control orCdkn2aUcp1KO mice under HFHS after intraperitoneal injection of insulin for insulin (ITT) tolerance tests (n= 6).lArea under the curve (AUC) analyses of (k).mEnergy expenditure of control (n= 5) orCdkn2aUcp1KO (n= 7) male mice fed a HFHS.nBody temperature of control orCdkn2aUcp1KO male mice during this experiment (n= 8).oImmunofluorescence staining of UCP1 and RFP in IGW from control orCdkn2aUcp1KO male mice. Scale bar, 50 μM.pQuantification of the percentage of RFP+ cells that express endogenous UCP1.qqPCR analysis of the mRNA expression of thermogenic genes in IGW from control orCdkn2aUcp1KO male mice (n= 6).rWestern blot analysis of UCP1 in IGW from control orCdkn2aUcp1KO male mice (n= 3).pvalues were determined by two-tailed Student’sttest. Data are expressed as means ± SEM. Primer sequences are available in Supplementary Table 2 . Oxygen consumption rate (OCR) analysis The oxygen consumption rate of beige adipocytes was measured by using a Seahorse XF96 Extracellular Flux Analyzer according to the manufacturer’s instructions. SVF cells were seeded on XF96 and induced to differentiate and maintain. The plate was subjected to a temperature-controlled (37 °C) extracellular analyzer at indicated time point. After measuring initial oxygen consumption rate (OCR), 4 μM oligomycin, 2 μM FCCP and 1 μM rotenone/actinomycin A were then sequentially added into the plate by automatic pneumatic injection. Data were analyzed by Seahorse Wave software. Basal respiration was calculated as [OCR initial – OCR R&A ]. The maximum respiration rate was computed as [OCR FCCP – OCR R&A ]. Measurement of mitochondrial DNA (mtDNA) The total DNA was isolated from beige adipocytes by using DNA isolation kit. mtDNA was amplified using primers specific for the mitochondrial cytochrome c oxidase subunit 2 (Cox2) gene and normalized to an intron of the nuclear-encoded Hbb (β-globin) gene as described before [54] . The primer sequences were listed in Supplementary Table 2 . RNA immunoprecipitation-qPCR (RIP-qPCR) RIP was performed by using a Dynabeads Protein A immunoprecipitation kit (Thermo Fisher Scientific) according to the manufacturer’s instructions. Briefly, mature adipocytes were lysed in lysis buffer (150 mM KCl, 10 mM HEPES, 2 mM EDTA, 0.5% NP-40, 0.5 mM DTT, protease inhibitor cocktail and RNase inhibitor) for 30 min at 4 °C. The lysates were centrifuged, and the supernatant was collected. A small aliquot of lysate was saved as input, and the remaining sample was incubated with Protein A magnetic beads conjugated with p16 INK4a , p19 ARF or IgG antibody at 4 °C for 4 h. Subsequently, the beads were washed with wash buffer and eluted in elution buffer. The input and immunoprecipitated RNAs were isolated by Tripure Isolation Reagent and reverse transcribed into cDNA. The fold enrichment was detected by qPCR. Co-immunoprecipitation (Co-IP) Co-IP was performed by using a Pierce crosslink magnetic IP/Co-IP kit (Thermo Fisher Scientific) according to the manufacturer’s instructions. Cells were rinsed with cold PBS, lysed in IP lysis buffer, cleared by centrifugation and protein concentration was estimated. A small aliquot of lysate was saved as input, and the remaining sample was incubated with Protein A magnetic beads conjugated with p16 INK4a , p19 ARF , BCL2L1 or IgG antibody at 4 °C overnight. Then, the beads were washed with wash buffer and eluted by heating in loading buffer. Immunoprecipitates and input were electrophoresed, transferred to PVDF membranes, and probed with the indicated antibodies. RNA stability assay RNA stability assay was performed as previously described [55] . Briefly, cells were treated with 5 µg/ml actinomycin D (Sigma-Aldrich) to inhibit global mRNA transcription. Samples were collected at the indicated time points. Total RNA was extracted for reverse transcription, and the levels of genes of interest were analyzed by qPCR. Human participants Study participants were recruited from the Bariatric and General Surgery Clinics at the University of Illinois Hospital. We enrolled twelve obese subjects (8 females and 4 males) who underwent laparoscopic gastric sleeve bariatric surgery and five lean healthy controls (3 females and 2 males) who underwent elective surgeries such as hernia repair and abdominal wall reconstruction. Subcutaneous adipose tissue samples were obtained during surgery. Adipose tissue samples were snap-frozen and stored for biological analyses. The age of the participants ranged from 21 to 47 years old. Exclusion criteria included chronic inflammatory diseases, chronic organ failure, autoimmune diseases, cancer of any type, current smoking, or current pregnancy. Subjects who were deemed eligible were informed about the study details, risks, and precautions taken to reduce this risk. All the study participants provided informed written consent. Physical characteristics, including body weight and body mass index (BMI), were measured. Total fat mass was assessed using dual x-ray absorptiometry (DXA; iDXA, General Electric Inc). Plasma concentrations of glucose were quantified in the fasting state as we previously described [56] . All protocols and procedures of the study followed the standards set by the latest version of the Declaration of Helsinki and were approved by the Institutional Review Board of The University of Illinois at Chicago (protocol code 2017-1125). 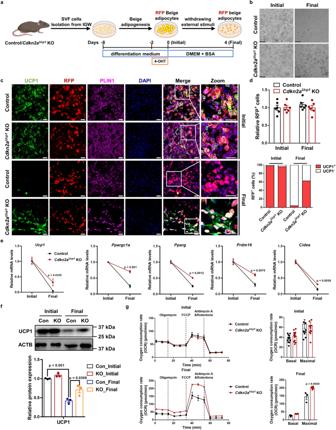Fig. 3:Cdkn2adeficiency promotes beige adipocyte maintenance in vitro. aSchematic illustration of the cellular system of beige adipocyte maintenance. SVF cells isolated from IGW of control orCdkn2aUcp1KO male mice were differentiated into beige adipocytes and treated with 4-OHT to induce gene deletion and RFP labeling. Then, external stimuli were withdrawn by changing the differentiation medium to DMEM containing 5% BSA for 4 days.bBright field images of control orCdkn2aUcp1KO beige adipocytes during beige adipocyte maintenance. Scale bar, 100 μM.cImmunofluorescence staining of UCP1 and RFP in control andCdkn2aUcp1KO beige adipocytes during beige adipocyte maintenance. Scale bar, 50 μM.dQuantification of RFP+ cells (upper panel) and the percentage of RFP+ cells that express endogenous UCP1 (lower panel) (n= 6).eqPCR analysis of the mRNA expression of thermogenic genes in control andCdkn2aUcp1KO beige adipocytes during beige adipocyte maintenance.fWestern blot analysis of UCP1 in control andCdkn2aUcp1KO beige adipocytes during beige adipocyte maintenance.gSeahorse analysis of oxygen consumption rates (OCR) in control andCdkn2aUcp1KO beige adipocytes during beige adipocyte maintenance (n= 12).pvalues were determined by two-tailed Student’sttest. Data are expressed as means ± SEM of triplicate tests. The details of population characteristics are listed in Supplementary Table 3 . Statistics and reproducibility All data are presented as mean ± SEM. Two-tailed unpaired Student’s t test (for comparison of two groups) or one‐way ANOVA followed by Tukey’s test (for comparison of three or more groups) were conducted using GraphPad Prism software. All experiments were repeated two or three times with representative data or images shown. 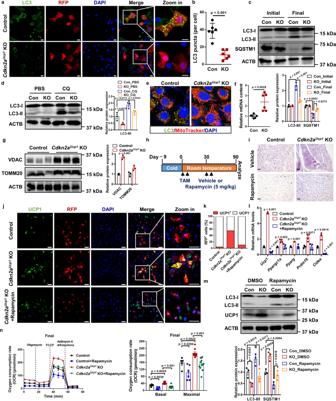Fig. 4:Cdkn2adeletion promotes beige fat maintenance by inhibiting autophagy. aImmunofluorescence staining of LC3 and RFP in control andCdkn2aUcp1KO beige adipocytes after withdrawing external stimuli. Scale bar, 10 μM.bQuantification of the number of LC3 puncta per cell (n= 6).cWestern blot analysis of LC3, SQSTM1 in control andCdkn2aUcp1KO beige adipocytes during beige adipocyte maintenance.dWestern blotting analysis of LC3 in control andCdkn2aUcp1KO beige adipocytes after withdrawing external stimuli and treated with or without 10 μM chloroquine (CQ).eImmunofluorescence staining of MitoTracker and LC3 in control andCdkn2aUcp1KO beige adipocytes after withdrawing external stimuli. Scale bar, 10 μM.fThe relative mtDNA copy number in control andCdkn2aUcp1KO beige adipocytes after withdrawing external stimuli.gWestern blot analysis of VDAC and TOMM20 in control andCdkn2aUcp1KO beige adipocytes after withdrawing external stimuli.hExperimental procedure. Two-month-old control andCdkn2aUcp1KO male mice were housed under cold conditions for 7 consecutive days to induce beige fat formation and then administered vehicle or 5 mg/kg rapamycin at room temperature for 90 days.iRepresentative H&E staining images of IGW from control orCdkn2aUcp1KO male mice treated with or without rapamycin. Scale bar, 100 μM.jImmunofluorescence staining of UCP1 and RFP in control andCdkn2aUcp1KO beige adipocytes treated with or without 10 nM rapamycin after withdrawing external stimuli. Scale bar, 50 μM.kQuantification of the percentage of RFP+ cells that express endogenous UCP1.lqPCR analysis of the mRNA expression of thermogenic genes in control andCdkn2aUcp1KO beige adipocytes treated with or without 10 nM rapamycin after withdrawing external stimuli (n= 3–4).mWestern blot analysis of UCP1 and LC3 in control andCdkn2aUcp1KO beige adipocytes treated with or without 10 nM rapamycin after withdrawing external stimuli.nSeahorse analysis of oxygen consumption rates (OCR) in control andCdkn2aUcp1KO beige adipocytes treated with or without 10 nM rapamycin after withdrawing external stimuli (n= 9–11).pvalues were determined by two-tailed Student’sttest. Data are expressed as means ± SEM of triplicate tests. 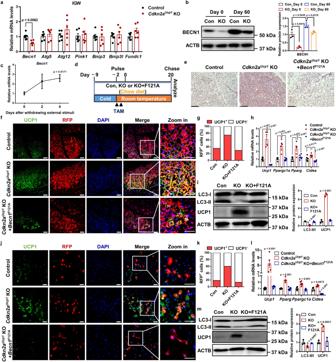Fig. 5:Cdkn2aregulates autophagy by positively mediatingBecn1expression in vivo and in vitro. aqPCR analysis of the mRNA expression of autophagy-related genes in IGW from control orCdkn2aUcp1KO male mice fed a HFHS (n= 6).bWestern blot analysis of BECN1 in IGW from control orCdkn2aUcp1KO male mice.cExpression profile ofBecn1during beige adipocyte maintenance.dExperimental procedure. Two-month-old control,Cdkn2aUcp1KO andCdkn2aUcp1KO +Becn1F121Amale mice were housed under cold conditions for 7 consecutive days to induce beige fat formation. Mice were then administered tamoxifen (TAM) and fed a chow diet at room temperature for 20 days.eRepresentative H&E staining images of IGW from control,Cdkn2aUcp1KO orCdkn2aUcp1KO +Becn1F121Amale mice after cold stimulus withdrawal. Scale bar, 100 μM.fImmunofluorescence staining of UCP1 in IGW from control,Cdkn2aUcp1KO orCdkn2aUcp1KO +Becn1F121Amale mice after cold stimulus withdrawal. Scale bar, 50 μM.gQuantification of the percentage of RFP+ cells that express endogenous UCP1.hqPCR analysis of the mRNA expression of thermogenic genes in IGW from control,Cdkn2aUcp1KO orCdkn2aUcp1KO +Becn1F121Amale mice after cold stimulus withdrawal (n= 6).iWestern blot analysis of UCP1 and LC3 in IGW from control,Cdkn2aUcp1KO orCdkn2aUcp1KO +Becn1F121Amale mice after cold stimulus withdrawal.jImmunofluorescence staining of UCP1 and RFP in control andCdkn2aUcp1KO beige adipocytes with or without hyperactive BECN1 after withdrawing external stimuli. Scale bar, 50 μM.kQuantification of the percentage of RFP+ cells that express endogenous UCP1.lqPCR analysis of the mRNA expression of thermogenic genes in control andCdkn2aUcp1KO beige adipocytes with or without hyperactive BECN1 after withdrawal of external stimuli (n= 4–6).mWestern blot analysis of UCP1 and LC3 in control andCdkn2aUcp1KO beige adipocytes with or without hyperactive BECN1 after withdrawing external stimuli.pvalues were determined by two-tailed Student’sttest. Data are expressed as means ± SEM of triplicate tests. 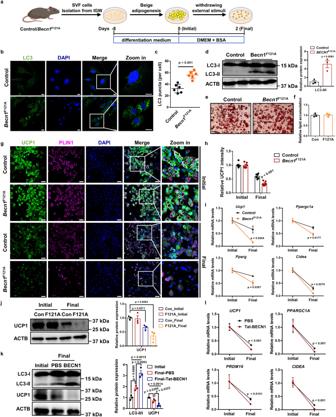Fig. 6: BECN1 does not influence beige biogenesis but accelerates the loss of beige adipocyte characteristics after withdrawal of external stimuli in vitro. aSchematic illustration of the cellular system of beige adipocyte maintenance. SVF cells isolated from IGW of control orBecn1F121Amale mice were differentiated into beige adipocytes. Then, external stimuli were withdrawn by changing the differentiation medium to DMEM containing 5% BSA for 2 days.bImmunofluorescence staining of LC3 in control andBecn1F121Abeige adipocytes. Scale bar, 10 μM.cQuantification of the number of LC3 puncta per cell (n= 6).dWestern blot analysis of LC3 in control andBecn1F121Abeige adipocytes.eOil red O staining of control andBecn1F121Abeige adipocytes before withdrawing external stimuli. Scale bar, 100 μM.fRelative lipid accumulation was quantified with a microplate spectrophotometer.gImmunofluorescence staining of UCP1 and PLIN1 in control andBecn1F121Abeige adipocytes during beige adipocyte maintenance. Scale bar, 50 μM.hQuantification of the percentage of UCP1-expressing cells (n= 6).iqPCR analysis of the mRNA expression of thermogenic genes in control andBecn1F121Abeige adipocytes during beige adipocyte maintenance.jWestern blot analysis of UCP1 in control andBecn1F121Abeige adipocytes during beige adipocyte maintenance.kWestern blot analysis of UCP1 and LC3 in human beige adipocytes treated with or without 5 μM Tat-BECN1 after withdrawal of external stimuli.lqPCR analysis of the mRNA expression of thermogenic genes in human beige adipocytes treated with or without 5 μM Tat-BECN1 after withdrawal of external stimuli.pvalues were determined by two-tailed Student’sttest. Data are expressed as means ± SEM of triplicate tests. p < 0.05 was considered statistically significant in all the experiments. 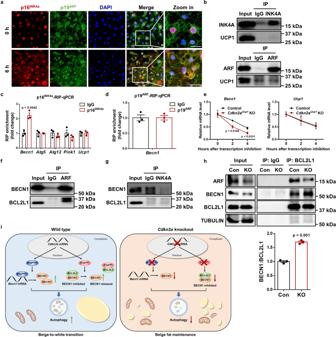Fig. 7:Cdkn2apositively regulatesBecn1expression by suppressing its mRNA decay and promotes BECN1-mediated autophagy by interacting with BCL2L1. aImmunofluorescence staining of p16INK4aand p19ARFdistribution during beige adipocyte maintenance.bWestern blot to confirm the immunoprecipitation of p16INK4aand p19ARFproteins.cRNA immunoprecipitation-qPCR (RIP-qPCR) analysis of the interaction ofBecn1,Atg5,Atg12,Pink1andUcp1transcripts with p16INK4ain beige adipocytes (n= 3).dRNA immunoprecipitation-qPCR (RIP-qPCR) analysis of the interaction of theBecn1transcript with p19ARFin beige adipocytes (n= 3).emRNA lifetimes ofBecn1andUcp1in control andCdkn2aUcp1KO beige adipocytes (n= 3).fCo-immunoprecipitation (Co-IP) analysis of the interaction between p19ARFand BECN1 or BCL2L1.gCo-IP analysis of the interaction between p16INK4aand BECN1 or BCL2L1.hCo-IP analysis of the interaction between BCL2L1 and BECN1 in control andCdkn2aUcp1KO beige adipocytes after withdrawing external stimuli (n= 3). Quantification of the BECN1/BCL2L1 ratio in the IP samples is shown in the right panel.iWorking model. In wild type cells, p16INK4aspecifically targetsBecn1mRNA and increases its expression by promoting mRNA stability, while p19ARFinteracts with BCL2L1 and releases BECN1, thereby enhancing autophagy and beige-to-white transition. Loss ofCdkn2adecreases the protein levels of p16INK4aand p19ARF, resulting in reduced expression and activity of BECN1, thereby inhibiting autophagy and promoting beige fat maintenance.pvalues were determined by two-tailed Student’sttest. Data are expressed as means ± SEM. 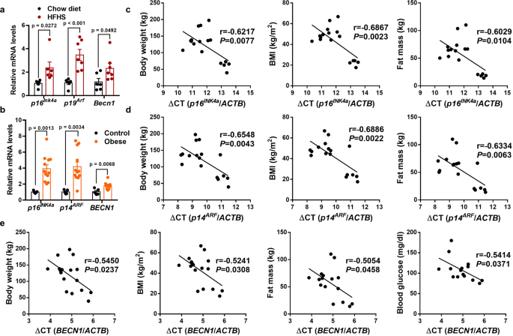Fig. 8:Cdkn2aandBecn1expression levels positively correlate with obesity in mice and humans. aqPCR analysis of the mRNA expression ofp16Ink4a,p19ArfandBecn1in IGW from male mice fed on chow diet or HFHS (n= 6–7).bqPCR analysis of the mRNA expression ofp16Ink4a,p14ArfandBecn1in subcutaneous WAT from obese and non-obese people (n= 5–12).cTwo-tailed Pearson’s correlation analysis ofp16INK4aexpression in human subcutaneous WAT and body weight, BMI or fat mass of 17 individuals.dTwo-tailed Pearson’s correlation analysis ofp14ARFexpression in human subcutaneous WAT and body weight, BMI or fat mass of 17 individuals.eTwo-tailed Pearson’s correlation analysis ofBECN1expression in human subcutaneous WAT and body weight, BMI, fat mass and blood glucose levels of 15–17 individuals.pvalues were determined by two-tailed Student’sttest. Data are expressed as means ± SEM. Reporting summary Further information on research design is available in the Nature Portfolio Reporting Summary linked to this article.